Spliced MDM2 isoforms promote mutant p53 accumulation and gain-of-function in tumorigenesis The tumour suppressor p53 is frequently mutated in tumours. Mutant p53 (Mutp53) proteins often gain new activities in promoting tumorigenesis, defined as gain-of-function (GOF). Mutp53 can accumulate to high levels in tumours, which promotes mutp53 GOF in tumorigenesis. The mechanism of mutp53 accumulation is poorly understood. Here we find that MDM2 isoforms promote mutp53 accumulation in tumours. MDM2 isoform B (MDM2-B), the MDM2 isoform most frequently over-expressed in human tumours, interacts with full-length MDM2 to inhibit MDM2-mediated mutp53 degradation, promoting mutp53 accumulation and GOF in tumorigenesis. Furthermore, MDM2-B overexpression correlates with mutp53 accumulation in human tumours. In mutp53 knock-in mice, a MDM2 isoform similar to human MDM2-B is overexpressed in the majority of tumours, which promotes mutp53 accumulation and tumorigenesis. Thus, overexpression of MDM2 isoforms promotes mutp53 accumulation in tumours, contributing to mutp53 GOF in tumorigenesis. This may be an important mechanism by which MDM2 isoforms promote tumorigenesis. Tumour suppressor p53 plays a crucial role in maintaining genomic stability and preventing tumour formation [1] , [2] . Disruption of normal p53 function is often a prerequisite for the development or progression of tumours. The p53 gene is mutated in ~50% of human tumours. The most common p53 mutation is single amino-acid substitution in the DNA-binding domain of the p53 protein. In addition to the loss of tumour-suppressive activity of wild-type p53 (wtp53), many tumour-associated mutant p53 (mutp53) proteins gain new functions independent of wtp53, defined as mutp53 gain-of-function (GOF), which enable them to contribute to malignant progression, including increased tumorigenesis and metastasis [3] , [4] . Mutp53 proteins often become stable and accumulate to high levels in human tumours, which is important for the execution of their GOF and contributes to more advanced tumours [3] , [5] , [6] . However, the regulation of mutp53, especially the mechanism for its accumulation in tumours, is poorly understood. E3 ubiquitin ligase MDM2 is a key negative regulator for p53. MDM2 forms a negative feedback loop with p53; as a p53-target gene, MDM2 can be transcriptionally induced by wtp53, which in turn degrades wtp53 through ubiquitination. MDM2 has been shown to retain the ability to bind to and degrade mutp53 (refs 7 , 8 ). Therefore, it was widely accepted that the accumulation of mutp53 in tumour cells is due to the inability of mutp53 to induce MDM2, which leads to the disruption of the MDM2-p53 negative feedback loop. However, this notion was challenged by recent studies showing that mutp53 accumulation was observed only in tumours but not in normal tissues in mice with knock-in of R172H or R270H mutp53 (equivalent to human R175H and R273H, respectively) [5] , [6] , [9] . Furthermore, MDM2 loss in these mice leads to mutp53 accumulation in normal tissues [9] . These findings suggest that MDM2 keeps mutp53 levels in check in normal tissues but not in tumour tissues, thus leading to mutp53 accumulation in tumours. These results strongly suggest that p53 mutations alone are insufficient for mutp53 accumulation, additional events occurring in tumours are required to release mutp53 from MDM2-mediated degradation, leading to mutp53 accumulation in tumours. MDM2 has multiple spliced isoforms. Some MDM2 isoforms, including MDM2 isoforms A, B and C, are frequently overexpressed in many types of human tumours. Furthermore, overexpression of these MDM2 isoforms occurs more frequently in high-grade tumours and is correlated with poor prognosis [10] , [11] , [12] , [13] , indicating a role of MDM2 isoforms in tumorigenesis. Some MDM2 isoforms, such as isoforms A, B and C, have been demonstrated to promote tumorigenesis [14] . However, the underlying mechanisms of MDM2 isoforms in tumorigenesis are not well understood. A common feature of majority of MDM2 isoforms is that they lack p53 binding domain but retain the C terminus, including the RING finger domain, to interact with full-length MDM2 (MDM2-FL) [13] , [15] . Previous studies reported that MDM2 isoforms increased wtp53 levels in in vitro cultured cells that express wtp53 (refs 16 , 17 ). However, the activation of wtp53 by MDM2 isoforms in cells could not explain the promoting effect of MDM2 isoforms on tumorigenesis. Here we tested the possibility that MDM2 isoforms overexpressed in tumours may interact with MDM2-FL and inhibit its function in degradation of mutp53, which in turn promotes mutp53 protein accumulation and enhances GOF of mutp53 in tumour cells. To test this hypothesis, we employed MDM2 isoform B (MDM2-B), the most common MDM2 isoform overexpressed in human tumours [13] , and investigated its effect on mutp53 protein accumulation and GOF in cells. We find that MDM2-B interacts with MDM2-FL and inhibits MDM2-FL binding to and degradation of mutp53. MDM2-B promotes mutp53 accumulation and mutp53 GOF in tumour growth and metastasis in mice. Furthermore, high expression levels of MDM2-B correlates with mutp53 accumulation in human tumours. Consistently, the majority of tumours in R172H mutp53 (p53 R172H/R172H ) knock-in mice express high levels of a MDM2 isoform similar to human MDM2-B in domain structure. This mouse MDM2 isoform promotes mutp53 accumulation in cells and promotes tumorigenesis in mice. These results demonstrate that overexpression of MDM2-B in tumours is an important mechanism for mutp53 accumulation in tumours, which contributes to mutp53 GOF in tumorigenesis. MDM2-B promotes mutp53 protein accumulation in cells MDM2-B is the most common MDM2 isoform highly expressed in human tumours [13] . MDM2-B lacks p53-binding domain, nuclear localization signal and nuclear export signal sequences, but retains the RING domain ( Fig. 1a ). p53 mutations have two major categories: DNA-contact mutations (including R248W and R273H tumour hotspot mutations) and conformational mutations (including R175H tumour hotspot mutation). To test our hypothesis that MDM2-B promotes mutp53 protein accumulation, we established cell lines with stable ectopic expression of R175H, R248W and R273H mutp53, respectively, in human p53-null lung cancer H1299 cells (H1299-R175H, H1299-R248W and H1299-R273H), and transfected MDM2-B-Flag expression vectors that express human MDM2-B with C-terminal Flag tag into these cell lines. As shown in Fig. 1b , ectopic expression of MDM2-B-Flag greatly increased the ectopic mutp53 protein levels in all of these cells. The effect of MDM2-B on endogenous mutp53 protein levels was also evaluated in a panel of human cancer cell lines. Ectopic expression of MDM2-B-Flag clearly increased endogenous mutp53 protein levels in both human colorectal HCT116 p53 R248w/− and breast T47D cells, which contain a single copy of p53 gene with R248W and L194F mutations, respectively ( Fig. 1c ). Ectopic expression of MDM2-B-Flag did not have an obvious effect on the RNA expression levels of mutp53 in above-mentioned cells ( Supplementary Fig. S1 ). The effect of MDM2-B upon wtp53 was also examined in H1299-HW24 cells, which express wtp53 under a tetracycline-regulated promoter [18] . Wtp53 is expressed with low concentrations of tetracycline and is maximally expressed in the absence of tetracycline. Supplementary Fig. S2 shows that ectopic expression of MDM2-B-Flag clearly increased wtp53 protein levels in H1299-HW24 cells with low concentrations (5 ng ml −1 ) of tetracycline, which is consistent with previous reports showing that MDM2 isoforms increase wtp53 levels in cells [16] , [17] . The effect of MDM2-B knockdown on mutp53 protein levels was further evaluated in HCT116 p53 R248w/− cells with stable ectopic expression of MDM2-B-Flag as well as T47D, liver Huh7 and colorectal DLD-1 cells that have high endogenous MDM2-B levels. Huh7 and DLD-1 cells contain a single copy of p53 gene with Y220C and S241F mutations, respectively. As shown in Fig. 1d–f , MDM2-B knockdown by siRNA specific for MDM2-B clearly decreased mutp53 protein levels in all these cells. To avoid off-target effects, two siRNA oligos against MDM2-B were used, and similar results were obtained. These results demonstrate that MDM2-B promotes mutp53 protein accumulation in cells. 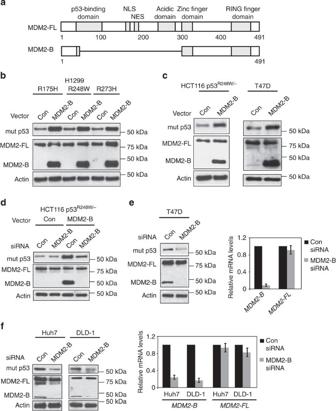Figure 1: MDM2-B promotes mutp53 protein accumulation in human cancer cells. (a) Schematic model showing the domain structure of MDM2-FL and MDM2-B. The amino acid residues are numbered. (b). Ectopic expression of MDM2-B-Flag by MDM2-B-Flag expression vectors (MDM2-B) increased mutp53 protein levels in H1299 cells with stable ectopic expression of mutp53 (R175H, R248W and R273H). (c) Ectopic expression of MDM2-B-Flag increased mutp53 protein levels in HCT116 p53R248w/−(left panel) and T47D (right panel) cells expressing endogenous mutp53. Con: Control. Inbandc, cells were transfected with MDM2-B-Flag expression vectors, and mutp53 protein levels were measured by western-blot assays at 24 h after transfection. (d) Knockdown of stably ectopically expressed MDM2-B-Flag in HCT116 p53R248w/−cells by siRNA specific against MDM2-B decreased mutp53 protein levels. (eandf) Knockdown of endogenousMDM2-Bby siRNA in T47D (e), Huh7 and DLD-1 (f) cells decreased the levels of endogenous mutp53 protein (left panel). Specific knock-down ofMDM2-Bbut notMDM2-FLwas confirmed at the mRNA level by Taqman real-time PCR assays (right panel). The expression levels of MDM2-B and MDM2-FL were normalized with actin. Two different siRNA oligos were used in (d–f), and similar results were obtained. Data in panelseandfare presented as mean±s.d.,n=3. Figure 1: MDM2-B promotes mutp53 protein accumulation in human cancer cells. ( a ) Schematic model showing the domain structure of MDM2-FL and MDM2-B. The amino acid residues are numbered. ( b ). Ectopic expression of MDM2-B-Flag by MDM2-B-Flag expression vectors (MDM2-B) increased mutp53 protein levels in H1299 cells with stable ectopic expression of mutp53 (R175H, R248W and R273H). ( c ) Ectopic expression of MDM2-B-Flag increased mutp53 protein levels in HCT116 p53 R248w/− (left panel) and T47D (right panel) cells expressing endogenous mutp53. Con: Control. In b and c , cells were transfected with MDM2-B-Flag expression vectors, and mutp53 protein levels were measured by western-blot assays at 24 h after transfection. ( d ) Knockdown of stably ectopically expressed MDM2-B-Flag in HCT116 p53 R248w/− cells by siRNA specific against MDM2-B decreased mutp53 protein levels. ( e and f ) Knockdown of endogenous MDM2-B by siRNA in T47D ( e ), Huh7 and DLD-1 ( f ) cells decreased the levels of endogenous mutp53 protein (left panel). Specific knock-down of MDM2-B but not MDM2-FL was confirmed at the mRNA level by Taqman real-time PCR assays (right panel). The expression levels of MDM2-B and MDM2-FL were normalized with actin. Two different siRNA oligos were used in ( d – f ), and similar results were obtained. Data in panels e and f are presented as mean±s.d., n =3. Full size image MDM2-B inhibits MDM2-FL to bind to and degrade mutp53 MDM2-B loses the p53-binding domain but retains the RING domain that can bind to MDM2-FL (ref. 15 ) ( Fig. 1a ), raising the possibility that MDM2-B increases mutp53 protein levels through blocking MDM2-FL-mediated degradation of mutp53. MDM2-FL can degrade mutp53 protein; ectopic expression of MDM2-FL by MDM2-FL expression vectors decreased mutp53 protein levels, whereas knockdown of endogenous MDM2-FL by siRNA increased mutp53 protein levels in HCT116 p53 R248w/− and T47D cells ( Fig. 2a,b ). Similarly, ectopic expression of MDM2-FL decreased mutp53 protein levels in H1299-R175H, H1299-R248W and H1299-R273H cells ( Supplementary Fig. S3 ). These results demonstrate that MDM2-FL retains the ability to degrade mutp53 protein, which is consistent with the previous report [8] . These results raise the possibility that some regulatory mechanisms result in the selective compromise of MDM2-FL function in tumours, leading to mutp53 protein accumulation in tumours. We investigated whether MDM2-B inhibits the function of MDM2-FL to degrade mutp53. To this end, p53 −/− mdm2 −/− (2KO) mouse embryonic fibroblasts (MEFs) were transfected with mutp53 (R248W or R175H) expression vectors together with MDM2-FL and/or MDM2-B-Flag expression vectors. Ectopic expression of MDM2-FL greatly decreased mutp53 protein levels, whereas ectopic expression of MDM2-B-Flag did not decrease mutp53 protein levels in 2KO cells ( Fig. 2c ). Notably, MDM2-B inhibited MDM2-FL-mediated degradation of mutp53 protein; co-expression of MDM2-B-Flag and MDM2-FL did not result in the decrease of mutp53 levels in 2KO cells ( Fig. 2c ). The inhibitory effect of MDM2-B on MDM2-FL-mediated degradation of mutp53 was observed when the molar ratio of MDM2-FL versus MDM2-B-Flag transfected is 1:0.25, and reached 90% when the ratio of MDM2-FL versus MDM2-B-Flag is 1:0.5 ( Supplementary Fig. S4 ). Similar results were observed in HCT116 p53 R248w/− and H1299-R175H cells; ectopic expression of MDM2-B-Flag or knockdown of endogenous MDM2-FL by siRNA can both increase mutp53 protein levels. Notably, MDM2-B had no obvious effect on mutp53 protein levels in cells with knockdown of MDM2-FL by siRNA, which already have increased mutp53 protein levels ( Fig. 2d and Supplementary Fig. S5 ). These results demonstrate that MDM2-B inhibits the function of MDM2-FL to degrade mutp53, leading to mutp53 protein accumulation in cells. 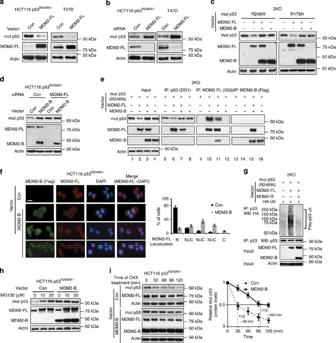Figure 2: MDM2-B promotes mutp53 accumulation through inhibition of MDM2-FL-mediated mutp53 degradation. (a) Ectopic expression of MDM2-FL down-regulated mutp53 protein levels in HCT116 p53R248w/−and T47D cells. mutp53 protein levels in cells were measured by western-blot assays at 24 h after transfection of MDM2-FL expression vectors. Con: Control. (b) Knockdown of endogenous MDM2-FL by siRNA increased mutp53 protein levels in HCT116 p53R248w/−and T47D cells. Two siRNA oligos were used, similar results were obtained. (c) MDM2-B inhibited MDM2-FL-mediated mutp53 degradation (R248W and R175H) in p53−/−mdm2−/−2KO MEFs. Indicated combination of expression vectors of MDM2-B-Flag (MDM2-B), MDM2-FL and mutp53 were co-transfected into cells. (d) Ectopic expression of MDM2-B-Flag increased mutp53 protein levels in HCT116 p53R248w/−but not in HCT116 p53R248w /−with knockdown of MDM2-FL by siRNA. Two siRNA oligos were used, similar results were obtained. (e) MDM2-B interacted with MDM2-FL and blocked the binding of MDM2-FL to mutp53(R248W) in 2KO cells as determined by IP assays. Antibodies used for IP: DO-1 for mutp53; 3G5, an antibody recognizing MDM2-FL but not MDM2-B; Flag for MDM2-B-Flag. (f) MDM2-B increased MDM2-FL protein localization in the cytoplasm as determined by IF staining in HCT116 p53R248w/−cells. Antibodies used for IF: 3G5 for MDM2-FL; Flag for MDM2-B-Flag. Nuclei were stained with DAPI. Scale bar: 20 μm. Lower panel: quantification of subcellular distribution of MDM2-FL in 200 cells for each experiment. Data are presented as mean±s.d. (n=3).P<0.005, χ2test. (g) MDM2-B decreased MDM2-FL-mediated mutp53 ubiquitination in 2KO cells. Cells were transfected with indicated combination of expression vectors of MDM2-B-Flag, MDM2-FL, mutp53 (R248W) and HA-ubiquitin (HA-Ub) for 24 h, then treated with proteasome inhibitor MG132 for 5 h. Mutp53 ubiquitination were determined by IP using DO-1 antibody followed by western-blot assays with an anti-HA or anti-p53 antibody. (h) Blocking proteasomal degradation by MG132 increased mutp53 levels in HCT116 p53R248w/−but not in HCT116 p53R248w/−with ectopic MDM2-B expression. (i) MDM2-B increased mutp53 protein half-life. HCT116 p53R248w/−cells with and without ectopic MDM2-B-Flag expression were treated with cycloheximide (CHX, 10 μg/ml) for indicated time before being collected for western-blot analysis. Data are presented as mean±s.d. (n=3). Figure 2: MDM2-B promotes mutp53 accumulation through inhibition of MDM2-FL-mediated mutp53 degradation. ( a ) Ectopic expression of MDM2-FL down-regulated mutp53 protein levels in HCT116 p53 R248w/− and T47D cells. mutp53 protein levels in cells were measured by western-blot assays at 24 h after transfection of MDM2-FL expression vectors. Con: Control. ( b ) Knockdown of endogenous MDM2-FL by siRNA increased mutp53 protein levels in HCT116 p53 R248w/− and T47D cells. Two siRNA oligos were used, similar results were obtained. ( c ) MDM2-B inhibited MDM2-FL-mediated mutp53 degradation (R248W and R175H) in p53 −/− mdm2 −/− 2KO MEFs. Indicated combination of expression vectors of MDM2-B-Flag (MDM2-B), MDM2-FL and mutp53 were co-transfected into cells. ( d ) Ectopic expression of MDM2-B-Flag increased mutp53 protein levels in HCT116 p53 R248w/− but not in HCT116 p53 R248w /− with knockdown of MDM2-FL by siRNA. Two siRNA oligos were used, similar results were obtained. ( e ) MDM2-B interacted with MDM2-FL and blocked the binding of MDM2-FL to mutp53(R248W) in 2KO cells as determined by IP assays. Antibodies used for IP: DO-1 for mutp53; 3G5, an antibody recognizing MDM2-FL but not MDM2-B; Flag for MDM2-B-Flag. ( f ) MDM2-B increased MDM2-FL protein localization in the cytoplasm as determined by IF staining in HCT116 p53 R248w/− cells. Antibodies used for IF: 3G5 for MDM2-FL; Flag for MDM2-B-Flag. Nuclei were stained with DAPI. Scale bar: 20 μm. Lower panel: quantification of subcellular distribution of MDM2-FL in 200 cells for each experiment. Data are presented as mean±s.d. ( n =3). P <0.005, χ 2 test. ( g ) MDM2-B decreased MDM2-FL-mediated mutp53 ubiquitination in 2KO cells. Cells were transfected with indicated combination of expression vectors of MDM2-B-Flag, MDM2-FL, mutp53 (R248W) and HA-ubiquitin (HA-Ub) for 24 h, then treated with proteasome inhibitor MG132 for 5 h. Mutp53 ubiquitination were determined by IP using DO-1 antibody followed by western-blot assays with an anti-HA or anti-p53 antibody. ( h ) Blocking proteasomal degradation by MG132 increased mutp53 levels in HCT116 p53 R248w/− but not in HCT116 p53 R248w/− with ectopic MDM2-B expression. ( i ) MDM2-B increased mutp53 protein half-life. HCT116 p53 R248w/− cells with and without ectopic MDM2-B-Flag expression were treated with cycloheximide (CHX, 10 μg/ml) for indicated time before being collected for western-blot analysis. Data are presented as mean±s.d. ( n =3). Full size image Co-immunoprecipitation assays showed that MDM2-B inhibited the interaction of MDM2-FL with mutp53 in 2KO cells transfected with mutp53 (R248W or R175H), MDM2-FL and/or MDM2-B-Flag. MDM2-FL readily interacted with mutp53 and MDM2-B ( Fig. 2e and Supplementary Fig. S6a ). The interaction of MDM2-FL with MDM2-B was also observed in H1299-R175H cells with ectopic expression of MDM2-B-Flag ( Supplementary Fig. S6b ). No interaction between MDM2-B and mutp53 was observed (lanes 8 and 16 in Fig. 2e ). Notably, co-expression of MDM2-B-Flag clearly decreased the interaction of MDM2-FL with mutp53 (lanes 7 and 11 in Fig. 2e and lane 7 in Supplementary Fig. S6a ). MDM2-B lacks nuclear localization signal, which mediates the process of importing target proteins into the nucleus ( Fig. 1a ). Indeed, MDM2-B was predominantly localized in the cytoplasm in 2KO cells transfected with MDM2-B-Flag ( Supplementary Fig. 7 ). It was reported that in cells that express wtp53, MDM2-B can bind to MDM2-FL in cytoplasm and reduces the localization of MDM2-FL in the nucleus, where MDM2-FL binds to wtp53 [16] . It is possible that the interaction of MDM2-B with MDM2-FL may reduce the localization of MDM2-FL in the nucleus, which in turn frees mutp53 from MDM2-FL binding and thereby leads to mutp53 protein accumulation. Indeed, while MDM2-FL was predominantly localized in the nucleus of HCT116 p53 R248w/− cells, ectopic expression of MDM2-B-Flag clearly increased the cytoplasmic localization of MDM2-FL in the cells as determined by immunofluorescence (IF) staining assays ( Fig. 2f ). Recent studies have also reported that the MDM2 RING domain forms dimers and oligomers in cells; using chemical crosslinking assays to link interacting proteins in cell lysates, a large fraction of MDM2-FL protein can be crosslinked into the high-molecular weight protein in H1299 cells [19] , [20] . Furthermore, the dimerization and oligomerization of MDM2-FL is needed for efficient p53 polyubiquitination; disruption of MDM2-FL dimerization and oligomerization can reduce the efficiency of p53 ubiquitination [19] , [20] . Consistent with previous reports, employing chemical crosslinking assays to link interacting proteins, a large fraction of MDM2-FL protein was crosslinked into the high-molecular weight protein in HCT116 p53 R248w/- cells ( Supplementary Fig. S8 ). Notably, the fraction of MDM2-FL protein crosslinked into high-molecular weight was greatly reduced in HCT116 p53 R248w/− cells with ectopic expression of MDM2-B, in which a significant amount of MDM2-FL-MDM2-B complex was observed ( Supplementary Fig. S8 ). This observation suggests that MDM2-B inhibits the dimerization/oligomerization of MDM2-FL, which is necessary for efficient ubiquitination of mutp53 by MDM2-FL. Consistently, MDM2-B reduced MDM2-FL-mediated ubiquitination of mutp53 in cells as determined by in viv o ubiquitination assays in 2KO cells ( Fig. 2g ). As an E3 ubiquitin ligase, MDM2-FL ubiquitinates p53 for proteasomal degradation [21] . Blocking proteasomal degradation by MG132, a proteasomal inhibitor, increased mutp53 protein levels in HCT116 p53 R248w/− and H1299-R175H cells ( Fig. 2h and Supplementary Fig. S9a ). Interestingly, MG132 had very limited effect on mutp53 protein levels in cells with ectopic MDM2-B-Flag expression ( Fig. 2h and Supplementary Fig. S9a ), indicating that MDM2-B inhibits the function of MDM2-FL in ubiquitination and degradation of mutp53. Furthermore, ectopic expression of MDM2-B-Flag significantly increased the half-life of mutp53 protein in HCT116 p53 R248w/− and H1299-R175H cells ( Fig. 2i and Supplementary Fig. S9b ). These results demonstrate that MDM2-B interacts with MDM2-FL, and inhibits MDM2-FL binding to and degradation of mutp53 protein, leading to increased half-life of mutp53 protein and its accumulation in cells. MDM2-B promotes mutp53 GOF in tumour growth and metastasis Promoting tumour cell proliferation and metastasis are the main GOF of mutp53 (refs 22 , 23 , 24 , 25 ). Here we found that MDM2-B promotes GOF of mutp53 in promoting tumour growth and metastasis. Stable ectopic expression of MDM2-B-Flag in HCT116 p53 R248w/− cells significantly promoted the growth of xenograft tumours in nude mice compared with control cells transfected with empty vectors ( P =0.008, ANOVA followed by Student’s t -test) ( Fig. 3a,b ). Results from both western-blot assays and immunohistochemistry (IHC) staining showed that MDM2-B-Flag expression resulted in mutp53 protein accumulation in HCT116 p53 R248w/− tumours ( Fig. 3c,d ). This promoting effect of MDM2-B on tumour growth is largely mutp53-dependent, since this effect was largely abolished in xenograft tumours formed by HCT116 p53 −/− ( Fig. 3a,b ). Furthermore, this promoting effect of MDM2-B on tumour growth is mediated by MDM2-FL, since knockdown of MDM2-FL largely abolished this effect ( Fig. 3e ). 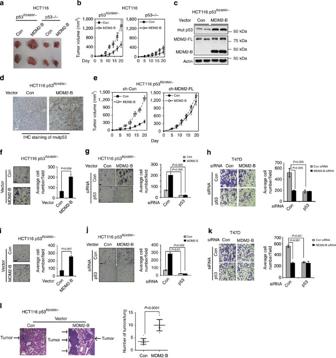Figure 3: MDM2-B increases mutp53 GOF in tumour growth and metastasis. (aandb) MDM2-B promoted xenograft tumour growth in a largely mutp53-dependent manner. BALB/c nude mice were inoculated (s.c.) with HCT116 p53R248w/−and HCT116 p53−/− cells with ectopic expression of MDM2-B-Flag (MDM2-B) or control cells transfected with control vectors (Con). (a) A representative image of xenograft tumours. (b) Growth curves of xenograft tumours. Tumour volumes are presented as mean±s.d.,n=10/group.P<0.01 Con versus MDM2-B in HCT116 p53R248w/−xenograft tumours, ANOVA, followed by Student’st-test. (candd) MDM2-B promoted mutp53 accumulation in HCT116 p53R248w/−xenograft tumours as determined by Western-blot assays (c) and IHC staining (d). Scale bar: 20 μm. (e) Knockdown of MDM2-FL greatly reduced the promoting effect of MDM2-B on the growth of HCT116 p53R248w/−xenograft tumours. Cells were transduced with shRNA vectors against MDM2-FL (sh-MDM2-FL) or control shRNA vectors (sh-Con). Two shRNA vectors were used, and similar results were obtained. Data are presented as mean±s.d.,n=10/group. (f–h) Ectopic expression of MDM2-B-Flag (MDM2-B) promoted invasion of HCT116 p53R248w/−(fandg) and knockdown of endogenous MDM2-B by siRNA decreased invasion of T47D (h) cells as determined by trans-well assays in chambers coated with matrigel. Data are presented as mean±s.d. (n=3).P<0.01, Studentt-test. This promoting effect of MDM2-B on invasion was largely abolished when mutp53 was knocked down by siRNA in HCT116 p53R248w/−cells (g) and T47D cells (h). Two siRNA oligos were used, and similar results were obtained. (i–k) Ectopic expression of MDM2-B-Flag promoted migration of HCT116 p53R248w/−(iandj) and knockdown of MDM2-B decreased migration of T47D (k) cells as determined by trans-well assays. Data are presented as mean±s.d. (n=3).P<0.01, Studentt-test. The promoting effect of MDM2-B on migration was largely abolished when mutp53 was knocked down by siRNA in HCT116 p53R248w/−cells (j) and T47D cells (k). (l) MDM2-B promoted lung metastasis of HCT116 p53R248w/−in vivo. HCT116 p53R248w/−cells with stable ectopic expression of MDM2-B-Flag (MDM2-B) and their control cells (Con) were injected into nude miceviatail vein, and the number of lung metastatic tumours was determined after 6 weeks (n=10/group). Scale bar: 30 μm. Data are presented as mean±s.d.P<0.0001, Studentt-test. Figure 3: MDM2-B increases mutp53 GOF in tumour growth and metastasis. ( a and b ) MDM2-B promoted xenograft tumour growth in a largely mutp53-dependent manner. BALB/c nude mice were inoculated (s.c.) with HCT116 p53 R248w/− and HCT116 p53−/− cells with ectopic expression of MDM2-B-Flag (MDM2-B) or control cells transfected with control vectors (Con). ( a ) A representative image of xenograft tumours. ( b ) Growth curves of xenograft tumours. Tumour volumes are presented as mean±s.d., n =10/group. P <0.01 Con versus MDM2-B in HCT116 p53 R248w/− xenograft tumours, ANOVA, followed by Student’s t -test. ( c and d ) MDM2-B promoted mutp53 accumulation in HCT116 p53 R248w/− xenograft tumours as determined by Western-blot assays ( c ) and IHC staining ( d ). Scale bar: 20 μm. ( e ) Knockdown of MDM2-FL greatly reduced the promoting effect of MDM2-B on the growth of HCT116 p53 R248w/− xenograft tumours. Cells were transduced with shRNA vectors against MDM2-FL (sh-MDM2-FL) or control shRNA vectors (sh-Con). Two shRNA vectors were used, and similar results were obtained. Data are presented as mean±s.d., n =10/group. ( f – h ) Ectopic expression of MDM2-B-Flag (MDM2-B) promoted invasion of HCT116 p53 R248w/− ( f and g ) and knockdown of endogenous MDM2-B by siRNA decreased invasion of T47D ( h ) cells as determined by trans-well assays in chambers coated with matrigel. Data are presented as mean±s.d. ( n =3). P <0.01, Student t -test. This promoting effect of MDM2-B on invasion was largely abolished when mutp53 was knocked down by siRNA in HCT116 p53 R248w/− cells ( g ) and T47D cells ( h ). Two siRNA oligos were used, and similar results were obtained. ( i – k ) Ectopic expression of MDM2-B-Flag promoted migration of HCT116 p53 R248w/− ( i and j ) and knockdown of MDM2-B decreased migration of T47D ( k ) cells as determined by trans-well assays. Data are presented as mean±s.d. ( n =3). P <0.01, Student t -test. The promoting effect of MDM2-B on migration was largely abolished when mutp53 was knocked down by siRNA in HCT116 p53 R248w/− cells ( j ) and T47D cells ( k ). ( l ) MDM2-B promoted lung metastasis of HCT116 p53 R248w/− in vivo . HCT116 p53 R248w/− cells with stable ectopic expression of MDM2-B-Flag (MDM2-B) and their control cells (Con) were injected into nude mice via tail vein, and the number of lung metastatic tumours was determined after 6 weeks ( n =10/group). Scale bar: 30 μm. Data are presented as mean±s.d. P <0.0001, Student t -test. Full size image Both invasion and migration are critical steps for tumour metastasis. HCT116 p53 R248w/− cells displayed increased invasion and migration abilities compared with HCT116 p53−/− cells in vitro as determined by trans-well assays ( Supplementary Fig. S10a,b ), demonstrating that mutp53 promotes invasion and migration of tumour cells, which is consistent with previous reports [24] , [25] . Notably, ectopic expression of MDM2-B-Flag greatly promoted invasion and migration of HCT116 p53 R248w/− cells ( Fig. 3f,i ). The promoting effects of MDM2-B on invasion and migration were much less pronounced in HCT116 p53 R248w/− cells with knockdown of mutp53 ( Fig. 3g,j ) or HCT116 p53−/− cells ( Supplementary Fig. S11a,b ). Consistently, knockdown of endogenous MDM2-B clearly decreased invasion and migration of T47D cells but not T47D cells with knockdown of mutp53 ( Fig. 3h,k ). These results indicate that MDM2-B promotes invasion and migration of tumour cells in vitro in a largely mutp53-dependent manner. The effect of MDM2-B on mutp53 GOF in metastasis was further investigated in vivo . Tail vein injection of HCT116 p53 R248w/− and HCT116 p53−/− cells can form lung metastatic tumours in nude mice. Ectopic expression of MDM2-B-Flag in HCT116 p53 R248w/− significantly increased the number of lung metastatic tumours ( Fig. 3l , P <0.0001, Student’s t -test). This promoting effect of MDM2-B on lung metastasis is largely mutp53-dependent since this effect was much less pronounced in HCT116 p53−/− cells ( Supplementary Fig. S12 ). These results demonstrate that MDM2-B promotes GOF of mutp53 protein, including tumour growth and metastasis. MDM2-B enhances the inhibitory effect of mutp53 on p63 and p73 One important mechanism of mutp53 GOF in tumorigenesis is the ability of mutp53 to bind to and inactivate p53 family members, p63 and p73 (refs 6 , 26 , 27 ). The transactivation isoforms of p63 and p73 can bind to the p53 DNA-binding elements in many p53-regulated genes, and therefore have partial functional overlap with p53. For instance, p53-regulated genes DDB2 and p21 can be transcriptionally activated by TAp63 and TAp73, respectively [28] , [29] . Luciferase reporter plasmids containing a p53-binding element in DDB2 or p21 promoter were employed to investigate whether MDM2-B enhances the inhibitory effect of mutp53 on transcriptional activities of p63 and p73 in H1299 cells. Luciferase reporter assays showed that mutp53 (R248W) decreased the transcriptional activities of TAp63 and TAp73 ( Supplementary Fig. S13a,b ). This effect of mutp53 was abolished by expression of MDM2-FL, which degrades mutp53, but reappeared when MDM2-B-Flag and MDM2-FL were co-expressed in cells ( Supplementary Fig. S13a,b ). Similarly, mutp53 (R248W) decreased the transcriptional induction of endogenous DDB2 and p21 by TAp63 and TAp73; respectively, in H1299 cells as examined by Taqman real-time PCR ( Supplementary Fig. S13c,d ). This effect of mutp53 was largely abolished by expression of MDM2-FL, but reappeared when MDM2-B-Flag and MDM2-FL were co-expressed in cells ( Supplementary Fig. S13c,d ). These data demonstrate that MDM2-B enhances the inhibitory effect of mutp53 on transcriptional activities of p63 and p73 through inhibition of the function of MDM2-FL in degradation of mutp53, which could be an important mechanism by which MDM2-B promotes mutp53 GOF. Overexpression of a MDM2 isoform in p53 R172H/R172H tumours Mouse MDM2 isoforms similar to human MDM2-B in structure, which lack p53-binding domain but retain RING finger domain, have been identified in mouse tumours, including B-cell lymphomas from Eμ-Myc transgenic mice and sarcomas from MDM2-overexpression mice [17] , [30] , [31] . We found that a MDM2 isoform similar to human MDM2-B in structure was overexpressed in tumours of p53 R172H/R172H mice, and correlated with mutp53 accumulation in tumours. p53 R172H/R172H mice mainly develop lymphomas in the spleen and thymus [6] . Using reverse transcription-PCR with a pair of primers in exons 1 and 12 that contains the stop codon, two major mouse MDM2 transcripts were detected in majority of tumour samples (12 out of 14 splenic lymphomas, 8 out of 10 thymic lymphomas), including the MDM2-FL and a MDM2 isoform similar to human MDM2-B in size ( Fig. 4a ). In contrast, this MDM2 isoform was not detected in normal spleen and thymus tissues of p53 R172H/R172H mice. This result was confirmed by Taqman real-time PCR and western-blot assays at RNA and protein levels, respectively ( Fig. 4b,c ). Previous reports showed that majority of tumours (~80%) from p53 R172H/R172H mice had increased mutp53 protein levels [6] , [9] . Similarly, mutp53 levels were low in normal tissues but increased substantially in all p53 R172H/R172H tumours we examined ( n =14 for splenic lymphomas, n =10 for thymic lymphomas) ( Fig. 4c ). DNA sequencing analysis revealed that the mouse MDM2 isoform overexpressed in p53 R172H/R172H tumours lacks exons 3–7 and 5′ 57 bases in exon 8, including the region coding for p53 binding domain, which is similar to human MDM2-B ( Fig. 4d ). Ectopic expression of this mouse MDM2 isoform in 2KO cells confirmed at the protein level that this MDM2 isoform expressed at the size corresponding to the protein overexpressed in tumours from p53 R172H/R172H mice ( Supplementary Fig. S14 ). Ectopic expression of this mouse MDM2 isoform in H1299-R175H, HCT116 p53 R248w/− as well as in p53 R172H/R172H MEF cells clearly led to mutp53 accumulation ( Fig. 4e ). The promoting effect of mouse MDM2 isoform on mutp53 accumulation is achieved mainly through inhibition of MDM2-FL function to degrade mutp53; while MDM2-FL expression decreased mutp53 levels in 2KO cells, co-expression of this mouse MDM2 isoform and MDM2-FL did not decrease mutp53 protein levels in 2KO cells ( Fig. 4f ). Furthermore, stable ectopic expression of this mouse MDM2 isoform in HCT116 p53 R248w/− cells significantly promoted the growth of xenograft tumours in nude mice compared with control cells transfected with control empty vectors ( P =0.01, ANOVA followed by Student’s t -test) ( Fig. 4g ). This promoting effect of mouse MDM2 isoform is largely mutp53-dependent since this effect was much less pronounced in xenograft tumours formed by HCT116 p53−/− ( Fig. 4g ). These results demonstrate that consistent with human MDM2-B, this mouse MDM2 isoform plays an important role in promoting mutp53 accumulation and GOF in tumours. 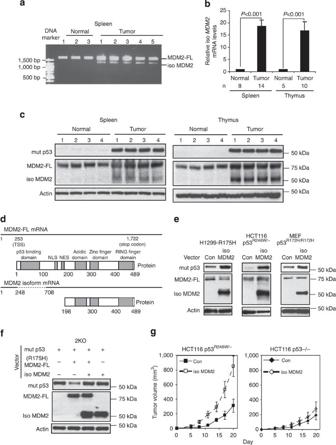Figure 4: Over-expression of the MDM2 isoform in p53R172H/R172Htumours promotes mutp53 accumulation and tumorigenesis. (a) Increased mRNA levels of the MDM2 isoform similar to human MDM2-B in splenic lymphomas from p53R172H/R172Hmice compared with normal spleen tissues as analysed by reverse transcription-PCR. (b) Increased mRNA levels of the MDM2 isoform similar to human MDM2-B in splenic and thymic lymphomas from p53R172H/R172Hmice compared with normal spleen and thymus tissues as analysed by Taqman real-time PCR. Data are presented as mean±s.d.P<0.001, Studentt-test. Normal spleen:n=8; splenic lymphoma:n=14; normal thymus:n=5; thymic lymphoma:n=10. (c) Increased MDM2 isoform protein levels correlate with mutp53 accumulation in splenic (left) and thymic (right) lymphomas. (d) Schematic model showing the domain structure of mouse MDM2-FL and the MDM2 isoform similar to human MDM2-B which is over-expressed in p53R172H/R172Htumours. TSS: translation starting site. (e) Ectopic expression of the mouse MDM2 isoform (iso MDM2) promoted mutp53 accumulation in H1299-R175H (left), HCT116 p53R248w/−(middle) and p53R172H/R172HMEF (right) cells. Con: Control. Cells were transfected with mouse MDM2 isoform expression vectors, and mutp53 protein levels were measured by western-blot assays at 24 h after transfection. (f) The mouse MDM2 isoform inhibited MDM2-FL-mediated degradation of mutp53 (R175H) in 2KO cells. (g) The mouse MDM2 isoform promoted the growth of HCT116 p53R248w/−xenograft tumours (P=0.01, ANOVA, followed by Student’st-test) (left panel). This promoting effect was largely abolished in HCT116 p53−/− xenograft tumours (right panel). Tumour volumes are presented as mean±s.d.,n=10/group. Figure 4: Over-expression of the MDM2 isoform in p53 R172H/R172H tumours promotes mutp53 accumulation and tumorigenesis. ( a ) Increased mRNA levels of the MDM2 isoform similar to human MDM2-B in splenic lymphomas from p53 R172H/R172H mice compared with normal spleen tissues as analysed by reverse transcription-PCR. ( b ) Increased mRNA levels of the MDM2 isoform similar to human MDM2-B in splenic and thymic lymphomas from p53 R172H/R172H mice compared with normal spleen and thymus tissues as analysed by Taqman real-time PCR. Data are presented as mean±s.d. P <0.001, Student t -test. Normal spleen: n =8; splenic lymphoma: n =14; normal thymus: n =5; thymic lymphoma: n =10. ( c ) Increased MDM2 isoform protein levels correlate with mutp53 accumulation in splenic (left) and thymic (right) lymphomas. ( d ) Schematic model showing the domain structure of mouse MDM2-FL and the MDM2 isoform similar to human MDM2-B which is over-expressed in p53 R172H/R172H tumours. TSS: translation starting site. ( e ) Ectopic expression of the mouse MDM2 isoform (iso MDM2) promoted mutp53 accumulation in H1299-R175H (left), HCT116 p53 R248w/− (middle) and p53 R172H/R172H MEF (right) cells. Con: Control. Cells were transfected with mouse MDM2 isoform expression vectors, and mutp53 protein levels were measured by western-blot assays at 24 h after transfection. ( f ) The mouse MDM2 isoform inhibited MDM2-FL-mediated degradation of mutp53 (R175H) in 2KO cells. ( g ) The mouse MDM2 isoform promoted the growth of HCT116 p53 R248w/− xenograft tumours ( P =0.01, ANOVA, followed by Student’s t -test) (left panel). This promoting effect was largely abolished in HCT116 p53−/− xenograft tumours (right panel). Tumour volumes are presented as mean±s.d., n =10/group. Full size image MDM2-B levels correlate with mutp53 levels in human tumours The correlation between MDM2-B overexpression and mutp53 accumulation was further confirmed in human colorectal cancer samples ( n =100). MDM2-B mRNA expression levels were significantly increased in a large percentage of colorectal cancers as determined by Taqman real-time PCR assays in formalin-fixed and paraffin-embedded (FFPE) tissues ( Fig. 5a ). Results from western-blot assays confirmed that at the protein level the increased expression of a MDM2 isoform at the size corresponding to MDM2-B in colorectal cancers compared with their adjacent normal tissues in a subset of fresh frozen tissues (14 out of 25 colorectal cancers) ( Fig. 5b ). The molecular mechanisms underlying MDM2-B over-expression in tumours are unclear. Here we tested whether mutp53 plays any role in MDM2-B overexpression. Mutp53 was knocked down by siRNA in T47D cells, and the expression of MDM2-B was determined at both RNA and protein levels by Taqman real-time PCR and western-blot assays, respectively. As shown in Supplementary Fig. S15 , knockdown of mutp53 did not have an obvious effect on the expression levels of MDM2-B, which excludes the possibility that mutp53 induces the levels of MDM2-B in tumours. 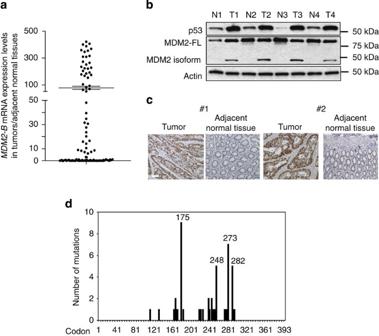Figure 5: MDM2-B over-expression correlates with mutp53 accumulation in human colorectal tumours. (a) MDM2-B mRNA levels were significantly increased in a large percentage of human colorectal cancers compared with adjacent normal tissues (n=100). Total RNA was prepared from FFPE colorectal cancers and their adjacent normal tissues. MDM2-B mRNA levels were determined by Taqman real-time PCR and normalized with actin. Data are presented as mean±s.d.,n=100/group. (b) Western-blot assays in a subset of fresh frozen human colorectal cancer tissues (n=25) confirmed the over-expression of a MDM2 isoform at the size corresponding to MDM2-B in human colorectal cancers. Representative images of western-blot assays showing the over-expression of the MDM2 isoform in tumours. T: tumours; N: adjacent normal tissues. (c) Representative images of p53 IHC staining in tissues. Scale bar: 30 μm. (d) The spectrum of p53 mutation identified by direct sequencing of exons 2–11 of thep53gene in human colorectal cancers. Figure 5: MDM2-B over-expression correlates with mutp53 accumulation in human colorectal tumours. ( a ) MDM2-B mRNA levels were significantly increased in a large percentage of human colorectal cancers compared with adjacent normal tissues ( n =100). Total RNA was prepared from FFPE colorectal cancers and their adjacent normal tissues. MDM2-B mRNA levels were determined by Taqman real-time PCR and normalized with actin. Data are presented as mean±s.d., n =100/group. ( b ) Western-blot assays in a subset of fresh frozen human colorectal cancer tissues ( n =25) confirmed the over-expression of a MDM2 isoform at the size corresponding to MDM2-B in human colorectal cancers. Representative images of western-blot assays showing the over-expression of the MDM2 isoform in tumours. T: tumours; N: adjacent normal tissues. ( c ) Representative images of p53 IHC staining in tissues. Scale bar: 30 μm. ( d ) The spectrum of p53 mutation identified by direct sequencing of exons 2–11 of the p53 gene in human colorectal cancers. Full size image p53 protein levels in FFPE tissues were determined by IHC assays, and a significant percentage of tumours showed p53 positive staining (66%; n =66) ( Fig. 5c ). Direct sequencing of the coding exons (exons 2–11) of p53 showed that 51% of tumour samples ( n =51) contain a mutation in the coding region of the p53 gene, whereas all of the normal tissues express wtp53 ( Fig. 5d ). Consistent with previous reports [32] , all of the p53 mutations that we identified in tumours ( n =51) are missense point mutations in the DNA-binding domain with codons 175, 248, 273 and 282 as mutational hotspots ( Fig. 5d ). Furthermore, almost all tumours containing mutp53 (50 out of 51) showed positive p53 staining. Notably, there is a clear correlation between MDM2-B overexpression and p53 accumulation. In all, 58% of tumours with p53-positive staining (38 out of 66) displayed significantly increased MDM2-B levels (over 4 to ~400-fold increase at the mRNA level) compared with adjacent normal tissues. Among these tumours, 79% of tumours (30 out of 38) contain p53 mutations. In tumours negative for p53 staining, which contain wtp53 in 33 tumours and mutp53 in 1 tumour, only 26% of tumours (9 out of 34) showed over four-fold increase of MDM2-B expression ( Table 1 ). These results demonstrate that MDM2-B overexpression is significantly correlated with accumulation of p53 protein, mainly mutp53 protein, in colorectal cancers ( P =0.006, χ 2 test). Table 1 Correlation between MDM2-B overexpression and p53 protein accumulation in human colorectal tumours. Full size table Many tumour-associated mutp53 proteins have been shown to exhibit GOF properties that promote tumour progression and metastasis [22] , [24] , [25] . Mutp53 proteins often accumulate to high levels in tumours, which results in the enhanced mutp53 GOF and is correlated with more advanced tumours [5] , [6] . However, the mechanisms by which mutp53 accumulates in tumours are not well understood. Results from this study provide clear evidence that overexpression of MDM2-B in tumours is an important mechanism to compromise the MDM2-FL activity in mutp53 degradation, which contributes to mutp53 accumulation in tumours. In this study, we demonstrated that MDM2-B binds to MDM2-FL and inhibits the function of MDM2-FL in degradation of mutp53, which leads to mutp53 accumulation and increased mutp53 GOF in tumour cells. Consistently, overexpression of a MDM2 isoform similar to human MDM2-B in structure was observed in majority of tumours in p53 R172H/R172H mice but not in normal tissues. This mouse MDM2 isoform promotes mutp53 accumulation in cells and tumour growth in a largely mutp53-dependent manner in mice. Our results further show that MDM2-B overexpression is significantly correlated with mutp53 accumulation in human colorectal tumours. Previous studies ever reported that MDM2 isoforms can increase wtp53 levels and function [16] , [17] . For instance, Evans et al . [16] reported that the binding of MDM2-B to MDM2-FL increases wtp53 activity. Dang et al . [17] reported similar observations with the mouse MDM2 isoforms. However, MDM2 isoforms are frequently overexpressed in tumours, and have been shown to promote tumorigenesis. The biological significance of the observation that MDM2 isoforms promote wtp53 protein accumulation and activity in cells is unclear. Our results that MDM2-B promotes mutp53 accumulation and its GOF in tumorigenesis highlights the biological significance of MDM2-B overexpression in tumours. In this study, we further investigated the mechanisms by which MDM2-B inhibits MDM2-FL binding to and degradation of mutp53. Results from this study showed that the interaction of MDM2-B and MDM2-FL increases the localization of MDM2-FL in the cytoplasm ( Fig. 2f ), thereby reducing the nuclear localization of MDM2-FL and decreasing the MDM2-FL binding to mutp53, which is mainly localized in the nucleus. Furthermore, the interaction of MDM2-B and MDM2-FL disrupts the dimerization and oligomerization of MDM2-FL, which is needed for efficient p53 ubiquitination by MDM2-FL ( Supplementary Fig. S8 ). Taken together, our results strongly suggest that MDM2-B may inhibit the function of MDM2-FL in degradation of mutp53 through two mechanisms. First, MDM2-B increases the cytoplasmic localization of MDM2-FL and thereby decreases MDM2-FL binding to mutp53 in the nucleus; second, MDM2-B disrupts the dimerization/oligomerization of MDM2-FL to reduce its E3 ligase activity towards mutp53. The mechanisms for MDM2-B over-expression in tumours are not well understood. Chandler et al . [33] reported that UV irradiation induced alternative splicing of the MDM2 gene, with MDM2-B as the predominant spliced MDM2 isoform, in several human cell lines. Results from this study suggest that mutp53 does not have an apparent effect on the expression levels of MDM2-B ( Supplementary Fig. S15 ). Future studies will further shed light on the underlying mechanisms for MDM2-B overexpression in tumours. In addition to MDM2, chaperone-associated ubiquitin ligase (CHIP) has been shown to target both wtp53 and mutp53 for degradation [34] , [35] , [36] , [37] . It has been suggested that some mutp53 proteins, especially those with conformational mutations, can interact with molecular chaperone Hsp90, which in turn inhibits the function of CHIP and MDM2-FL in mutp53 degradation [34] . Disruption of Hsp90-mutp53 interaction by siRNA or an Hsp90 inhibitor can liberate mutp53 and lead to CHIP- and MDM2-FL mediated mutp53 degradation [36] . A recent study by Li et al . [37] further demonstrated that suberoylanilide hydroxamic acid (SAHA), a histone deacetylase (HDAC) inhibitor, can inhibit HDAC6, an essential positive regulator of HSP90, which in turn releases mutp53 and promotes mutp53 degradation, resulting in preferential cytotoxicity for tumour cells expressing mutp53. Interestingly, a recent study showed that mutp53 protein can be induced by stress signals such as ionizing radiation and reactive oxygen species [38] . Considering that the levels and activities of wtp53 are regulated by many positive and negative regulators and different mechanisms in cells, the levels of mutp53 could be regulated by other mechanisms in addition to MDM2, CHIP and Hsp90. Future studies should further increase our understanding of the regulation of mutp53 and MDM2-B levels in cells. In summary, this study demonstrates that MDM2-B interacts with MDM2-FL and inhibits its function to degrade mutp53, which leads to mutp53 accumulation and increased mutp53 GOF in tumours. Thus, overexpression of MDM2-B is an important mechanism for mutp53 accumulation in tumours, which contributes to mutp53 GOF in tumorigenesis. Furthermore, mutp53 accumulation and resultant enhanced mutp53 GOF is an important mechanism by which MDM2-B promotes tumorigenesis. The role of MDM2-B in promoting the accumulation and GOF of mutp53 provides a rationale for new therapeutic strategies by targeting MDM2-B overexpression in tumours carrying mutp53. Cells and cell transfection Human H1299 (p53-null), T47D (mutp53), Huh7 (mutp53) and DLD-1 (mutp53) cells were obtained from ATCC. Human HCT116 p53 +/+ , HCT116 p53 –/– and HCT116 p53 R248w/− cells were generous gifts from Dr B. Vogelstein at Johns Hopkins University. Mouse p53 −/− mdm2 −/− double-knockout (2KO) embryonic fibroblasts were generous gifts from Dr Guillermina Lozano at M.D. Anderson Cancer Center. Human lung H1299-HW24 cell line that expresses wtp53 under the regulation of tetracycline was a generous gift from Dr Carol Prives at Columbia University [18] . p53 R172H/R172H MEFs were generated from p53 R172H/R172H mice as described previously [39] . In brief, MEFs were obtained from 13.5-day-old male and female embryos, and cultured at 37 °C in DMEM containing 10% fetal bovine serum supplemented with penicillin and streptomycin. Transfections of above-mentioned cells with plasmids or siRNA were performed by using Lipofectamine 2000 (Invitrogen). siRNA oligos against MDM2-FL and p53, respectively, were purchased from Integrated DNA Technologies. siRNA target MDM2-FL: 5′ AUGUGAAGAUGAAGGUUUCUCUUCCUG 3′; siRNA target p53: 5′ GACUCCAGUGGUAAUCUACUU 3′. Another set of pre-designed, functionally validated siRNA oligos against MDM2-FL (Cat#SI00300846) and p53 (Cat#SI02655170) were purchased from Qiagen. Two siRNA oligos against MDM2-B were designed at the splicing junction, which specifically target MDM2-B but not MDM2-FL; siRNA-1: 5′ GAGACCCUGGACUAUUGGA 3′; siRNA-2: 5′ GACCCUGGACUAUUGG 3′. Retroviral shRNA vectors against MDM2-FL purchased from Open Biosystems, Thermo Scientific (Cat# RHS4531-EG4193) were transduced into HCT116 p53 R248w/− and selected by puromycin. Cells were treated with various concentrations of proteasome inhibitor MG132 (Sigma) or cycloheximide (CHX) (Sigma) for various time periods before being harvested for further analysis. Construction of plasmids The pCMV-MDM2-B-Flag vector was cloned by inserting the MDM2-B DNA fragment from the pCDNA-MDM2-B expression vector (a generous gift from Dr Linda Harris at St Jude Children’s Research Hospital) into the pCMV-Flag vector (Sigma). Mouse MDM2 isoform detected in tumours was amplified by the following pair of primers: forward: 5′-CCGCTCGAGATGTGCAGCGGCGGCAGCA-3′, reverse: 5′-GGAATTCGCGTTGAAGTAAGTTAGCACAATCA-3′. The PCR products were cloned into the pCMV-Flag plasmid. Western-blot assays Standard western-blot assays were used to analyse the levels of protein. Anti-p53 (FL393; 1:1,000 dilution) (Santa Cruz), anti-MDM2 (2A10; 1:1,000 dilution) [40] , anti-Flag (1:10,000 dilution; Sigma) and anti–β-actin (1:20,000 dilution; Sigma) antibodies were used to determine the levels of total p53, MDM2 (including MDM2-FL and MDM2-B), MDM2-B-Flag and Actin, respectively. The full blots are shown in Supplementary Figs S16 and 17 . Immunoprecipitation assays For immunoprecipitation (IP) experiments, 1 × 10 6 2KO and H1299-R175H cells were transfected with different expression vectors, including mutp53 vector (1 μg), MDM2-FL vector (3 μg), and MDM2-B-Flag vector (3 μg). Cells were harvested at 24 h after transfection and lysed in NP-40 buffer. Anti-p53 (DO-1, 1:100 dilution; Santa Cruz), anti-MDM2 (3G5, 1:50 dilution) [40] , a MDM2 antibody recognizing p53 binding domain, which is missing in MDM2-B, and anti-Flag antibodies (1:100 dilution) were used to pull down mutp53, MDM2-FL and MDM2-B-Flag, respectively. IF staining assays IF staining was performed as previously described [41] . In brief, cells grown on slides were fixed with 4% paraformaldehyde for 30 min and treated with 0.5% Triton X-100 for 5 min, blocked with 1% bovine serum albumin for 30 min and stained with anti-MDM2 (3G5; 1:50 dilution) and anti-Flag (1:300 dilution) antibodies to detect MDM2-FL and MDM2-B-Flag, respectively. Slides were washed and then incubated with Alexa Fluor 555 Goat Anti-Mouse IgG (H+L) (Invitrogen) and Alexa Fluor 488 Goat Anti-Rabbit IgG (H+L) (Invitrogen). Nuclei were stained with 4′, 6-diamidino-2-phenylindole (DAPI; Vector). In vivo ubiquitination of p53 2KO cells (1 × 10 6 ) were transfected with different expression vectors, including mutp53 vector (1 μg), MDM2-FL vector (3 μg), MDM2-B-Flag vector (3 μg) and HA-ubiquitin vector (3 μg). At 24 h after transfection, cells were treated with MG132 (30 μM) for 5 h. Cells were then harvested and lysed in NP-40 buffer. The levels of mutp53 ubiquitination were determined by IP using DO-1 antibody (for mutp53) followed by western-blot assays with an anti-HA (1:1,000 dilution) or anti-p53 (1:1,000 dilution) antibody. Chemical crosslinking of proteins Chemical crosslinking of proteins was performed as previously described [20] . In brief, cells were lysed in NP-40 lysis buffer. Cell lysate containing 20 μg of protein was incubated with 0.02% glutaraldehyde for 20 min at 4 °C. The reaction was stopped by adding 2 × Laemmli SDS sample buffer and proteins were analysed by western-blot assays. Quantitative Taqman real-time PCR Total RNA from cells or mouse tissues were prepared by using an RNeasy kit (Qiagen). Total RNA from FFPE colorectal tumour sections was prepared by using a High Pure miRNA Isolation kit (Roche). cDNA was prepared by using a High Capacity cDNA Reverse Transcription Kit (Applied Biosystems). Human MDM2-B, MDM2-FL, p53, DDB2 and p21 primers, human and mouse β-actin primers were purchased from Applied Biosystems. Following primers and probe were used for Taqman real-time PCR assays for the mouse MDM2 isoform: forward: 5′-CGGATCACCGCGCTTCT-3′; reverse: 5′-TTCTGTCTCACTAATGGATCTCCTTCT-3′; probe: 5′-CCTCCAGACTGTCTACC-3′. The probe targets the splicing junction of the mouse MDM2 isoform. Taqman real-time PCR was done in triplicate with TaqMan PCR mixture (Applied Biosystems). The expression of genes was normalized with the β-actin gene. The specificity of MDM2-B and MDM2-FL primers were confirmed in 2KO cells transiently transfected with expression vectors of MDM2-FL or MDM2-B-Flag. The mRNA expression levels of MDM2-B, MDM2-FL and β-actin were determined by Taqman real-time PCR. The PCR products were analysed by agarose gel electrophoresis ( Supplementary Fig. S18 ). Luciferase reporter assays pGL3 reporter vectors containing the p53-binding element in DDB2 (pGL3-DDB2) or p21 (pGL3-p21) promoter were employed for luciferase reporter assays. H1299 cells were transfected with the combination of different expression vectors including mutp53, TAp63, TAp73, MDM2-FL and MDM2-B-Flag expression vectors, luciferase reporter vectors pGL2-DDB2 or pGL3-p21. pRL-SV40 vectors expressing Renilla luciferase were co-transfected as an internal control to normalize the transfection efficiency. The luciferase activities were measured at 24 h after transfection by using the Dual-Luciferase Reporter Assay system (Promega). Cell migration and invasion assays The transwell system (24 wells, 8 μM pore size, BD Biosciences) was employed for cell migration and invasion assays. For migration assays, 1–3 × 10 4 cells in 300 μl of FBS-free medium were seeded into upper chambers, and the lower chamber was filled with 750 μl medium supplemented with 10% FBS. For T47D cells, the lower chamber was filled with 1:1 mix of medium supplemented with 10% FBS and NIH 3T3 cell-conditioned medium. For matrigel invasion assay, transwell membranes were pre-coated with 50 μl Matrigel (BD Biosciences). After cells were cultured at 37 °C for 24 h, cells in the upper surface of the membrane were removed and cells on the lower surface were fixed with methanol and stained with crystal violet. The number of cell was counted in at least five randomly selected fields under an optical microscope. Xenograft tumorigenicity analysis The 7-week-old BALB/c nu/nu male athymic nude mice (Taconic) were employed for xenograft tumorigenicity analysis with the approval of the Institutional Animal Care and Use Committee of Robert Wood Johnson Medical School of Rutgers State University of New Jersey. Cells (5 × 10 6 in 0.2 ml PBS) were injected subcutaneously (s.c.) into nude mice. After injection, mice were examined and tumour volumes were measured three times/week for 3 weeks. Tumour volume=1/2 (length × width 2 ). Tumour samples were processed for routine histopathological examination. In vivo lung metastasis analysis For lung metastasis analysis, HCT116 p53 R248w/− and HCT116 p53−/− cells with stable ectopic expression of MDM2-B-Flag and control cells with stable transfection of control empty vectors (2 × 10 6 in 0.1 ml PBS) were injected into nude mice via tail vein. The mice were killed at 6 weeks after the inoculation and lungs were removed and fixed in formaldehyde. The number of lung metastatic tumours was counted under a dissecting microscope and confirmed by histopathological analysis. Animal protocols were approved by the Institutional Animal Care and Use Committee of Robert Wood Johnson Medical School of Rutgers State University of New Jersey. Detection of MDM2 isoforms in mouse tumours Total RNA was isolated from mouse normal and tumour tissues using an RNeasy kit (Qiagen). cDNA was prepared by using random primers and a Taqman reverse transcription kit (Applied Biosystems). A pair of primers was used to amplify MDM2 and its isoforms. The sequences of the primers are as following: exon 1 forward: 5′-CCGCTCGAGGCTTTGTTAACGGG-3′; exon 12: reverse: 5′-GGAATTCCTAGTTGAAGTAAGTT-3′. Tumour specimens Deidentified colorectal cancer tissues and their adjacent normal tissues ( n =100 for FFPE tissues; n =25 for fresh frozen tissues) were randomly collected from the database of The First Affiliated Hospital of Harbin Medical University (Harbin, China) from January 2001 to January 2010. None of the patients received pre-surgical chemotherapy. The use of human samples in this study has an IRB approval from the ethics committee of Harbin Medical University. Mutation detection of p53 in colorectal cancer tissues The mutation detection of the p53 gene was carried out by amplification of exons 2–11 from genomic DNA with 9 pairs of primers within flanking intron sequences and then direct sequencing of these fragments from both sides. The sequences of primers are listed in Supplementary Table S1 . IHC assays of p53 in tumours IHC staining for p53 was performed as previously described [42] . In brief, tissue sections were deparaffinized in xylene and rehydrated with ethanol. Tissue sections were then preincubated with 10% normal goat serum in PBS (pH 7.5) followed by incubation with anti-p53 antibody (DO-1, 1:100 dilution) for overnight at 4 °C. Tissue sections were then stained with biotinylated secondary antibody (Vector). Immunoreactivity was detected by using a Vectastain Elite ABC kit (Vector). Known positive controls were included in each experiment, and negative controls were obtained by omitting the primary antibody. Statistical analysis The data were expressed as mean±s.d. The differences in xenograft tumour growth among groups were analysed for statistical significance by ANOVA, followed by Student’s t -tests using a GraphPad Prism software. All other P -values were obtained using Student t -test or χ 2 test. Values of P <0.05 were considered to be significant. How to cite this article: Zheng, T. et al . Spliced MDM2 isoforms promote mutant p53 accumulation and gain-of-function in tumorigenesis. Nat. Commun. 4:2996 doi: 10.1038/ncomms3996 (2013).